Electrochemical generation of hydrogen peroxide from a zinc gallium oxide anode with dual active sites 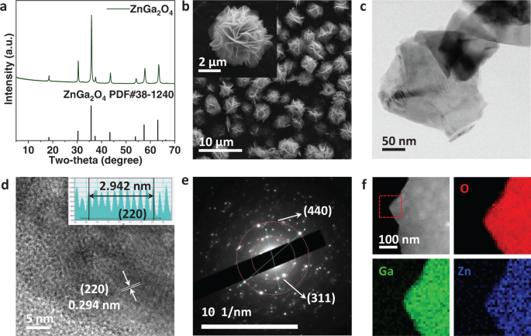Fig. 1: Morphological characterizations of ZnGa2O4. aX-ray diffraction pattern of the prepared ZnGa2O4.bSEM images of ZnGa2O4.cTEM image.dHRTEM image.ePolycrystalline electron diffraction pattern of ZnGa2O4.fScanning transmission electron microscopy electron energy loss spectroscopy (STEM-EELS) of the ZnGa2O4. Electrochemical water oxidation enables the conversion of H 2 O to H 2 O 2 . It holds distinct advantages to the O 2 reduction reaction, which is restricted by the inefficient mass transfer and limited solubility of O 2 in aqueous media. Nonetheless, most reported anodes suffer from high overpotentials (usually >1000 mV) and low selectivity. Electrolysis at high overpotentials often causes serious decomposition of peroxides and leads to declined selectivity. Herein, we report a ZnGa 2 O 4 anode with dual active sites to improve the selectivity and resist the decomposition of peroxides. Its faradaic efficiency reaches 82% at 2.3 V versus RHE for H 2 O 2 generation through both direct (via OH − ) and indirect (via HCO 3 − ) pathways. The percarbonate is the critical species generated through the conversion of bicarbonate at Ga-Ga dual sites. The peroxy bond is stable on the surface of the ZnGa 2 O 4 anode, significantly improving faradaic efficiency. Hydrogen peroxide (H 2 O 2 ) is a clean and valuable oxidant with wide applications in chemical synthesis [1] , [2] , energy technology [3] , [4] , [5] , and environmental remediation [6] , [7] , [8] . Currently, most H 2 O 2 is produced by an anthraquinone process [9] , which requires expensive Pd catalysts and produces a huge volume of organic waste [10] . Considerable efforts have been dedicated to producing H 2 O 2 in small-scale and more sustainable ways [11] , [12] , [13] , [14] . For example, the direct synthesis method (Eq. ( 1 )) has been developed using H 2 , O 2 , and noble metal catalysts in a liquid medium [15] , [16] , [17] . However, inert gases (N 2 or CO 2 ) are needed to dilute the reactant gases to eliminate the explosive risk. H_2+O_2→H_2O_2 G_298K^o=-135.9 kJ mol^-1. (1) The inherent limitations of Eq. ( 1 ), including the low solubility and inefficient mass transfer of gas reactants, the requirement for high-valued H 2 , and the safety concerns, have motivated researchers toward more feasible production routes. Alternatively, H 2 O 2 generation can start with abundant feedstocks such as water and oxygen. The main-stream O 2 reduction reaction (ORR, Eq. ( 2 )) has been demonstrated on some noble metals or carbon-based catalysts [12] , [18] , [19] , [20] . O_2+2H^++2e^-⇌H_2O_2 E^0=+ 0.68V versus RHE. (2) However, 2 electron-ORR is subjected to low solubility (8 mg L −1 , 1 atm, 25 °C) and low diffusion coefficient of O 2 in water (2.1 × 10 −5 cm −2 s −1 ) [21] . The O 2 reduction way requires continuous feeding of O 2 or air to the cathode surface, which brings extra production costs. Though these mass transfer problems can be overcome by gas diffusion electrodes (GDEs), it has been widely recognized that the effectiveness of GDEs suffers from a common flooding effect [22] , [23] , i.e. electrolyte penetration into the porous GDE. By contrast, the kinetics of the water oxidation reaction (WOR, Eq. ( 3 )) would not be limited by the mass transfers of reactants. A high faradaic current density can therefore be attained. 2e-WOR can meet the onsite demand for H 2 O 2 in O 2 -deficient environments, such as bacteria-contaminated water bodies [8] , which represents an obvious advantage over other production methods that require O 2 . Besides, the WOR reaction can be coupled with reduction reactions at the cathode, including hydrogen evolution, ORR, and CO 2 reduction reaction, to fully utilize the half-cell reactions. 2H_2O⇌H_2O_2+2H^++2e^- E^0=+ 1.76V versus RHE. (3) There are still several challenges to use the 2e-WOR technique effectively. First, the faradaic efficiency (FE) of H 2 O 2 is low, especially at low overpotentials. Though some metal oxides and carbon-based catalysts have been reported for 2e-WOR [7] , [24] , [25] , [26] , most of these catalysts usually require overpotentials larger than 1000 mV to achieve a satisfactory FE. High overpotentials required for anodes will reduce the overall energy efficiency of the electrocatalytic cells. Recently, progress has been made in lowering the overpotential by fabricating new anodes, for example, H 2 O 2 FE reaching 66% on CP/PTFE with an overpotential of 640 mV [27] , and reaching 72% on CuWO 4 with an overpotential of 740 mV [28] . Moreover, the electrochemical stability (including stable generation rate and FE) and the structural stability are also challenging because of the highly oxidative environment. Nevertheless, the main goal of 2e-WOR research is still to develop efficient and stable anodes with high selectivity at low overpotentials. 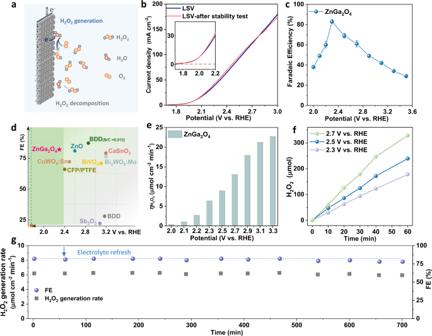Fig. 2: Activity and stability of H2O2generation on ZnGa2O4anode. aScheme of the electrochemical H2O2production on anodes through a water oxidation reaction.bLSV curves recorded in 2 M KHCO3before and after a stability test. The scan rate is 5 mV s−1.cH2O2FE of the prepared ZnGa2O4anode at different potentials in 2 M KHCO3electrolyte (Error bars represent the standard deviation of three independent measurements).dThe FE of typically reported anodes including ZnO25, boron-doped diamond (BDD)33, BDD (B/D ratio = 0.012)39BiVO438, CaSnO324, Bi2WO6:Mo7, and Sb2O326for H2O2generation in bicarbonate/carbonate electrolyte for comparison. The orange star represents the thermodynamic potential of 2e-WOR.eThe H2O2generation rate on the ZnGa2O4anode at different potentials.fThe accumulated amount of H2O2in 60 min-electrolysis under different applied potentials, (50 mL electrolyte, electrode area = 0.5 cm2).gThe FE and generation rate of H2O2on ZnGa2O4anode with an applied bias of 2.3 V versus RHE in 700 minutes. The electrolyte was periodically replaced. For the studies of anodic H 2 O 2 production, the performance of anodes is usually evaluated in bicarbonate electrolytes (usually 2 M KHCO 3 ) since many studies have demonstrated the promotion effect [7] , [29] , [30] , [31] and the stabilizing effect [32] of bicarbonate toward anodic H 2 O 2 production. A critical but often ignored issue is the decomposition of H 2 O 2 during long-time water oxidation. For example, the H 2 O 2 generation rate declines after passing 100 C for FTO/BiVO 4 [29] , after 3 h-electrolysis for FTO/CaSnO 3 [24] , after 3 h-reaction for FTO/Sb 2 O 3 [26] , after for 1000 s for boron-doped diamond [33] , and after 150 min-electrolysis for CaSnO3@CF [34] . A similar observation was also reported on C, N-codoped TiO 2 in 0.05 M Na 2 SO 4 after 2 h-electrolysis [35] . In these reports (details in Table S1 ), the H 2 O 2 concentration reaches a saturation level and does not increase further. Factors associated with the concentration plateau are considered inseparable from the instability of H 2 O 2 during electrolysis but await in-depth investigation. Typically, the decomposition of H 2 O 2 can occur either on the anode surface or in the bulk electrolyte. Firstly, the oxidation of H 2 O 2 occurs thermodynamically at a relatively low potential of 0.68 V versus RHE (reverse of Eq. ( 2 )). Therefore, there is a need to develop anode materials with sluggish H 2 O 2 oxidation kinetics. Otherwise, electrolysis at high potentials would cause severe H 2 O 2 electro decomposition on the anode surface. Secondly, anode material may induce H 2 O 2 decomposition, and the decomposition rate is material-dependent [26] , [30] , [36] . For instance, the current density associated with the electro decomposition of H 2 O 2 on BiVO 4 is estimated to be ~11 μA cm −2 mM H 2 O 2 in 0.5 M KHCO 3 electrolyte [30] , which is an order of magnitude smaller than that on Pt surface in phosphate buffer [36] . Thirdly, H 2 O 2 can undergo disproportionation (Eq. ( 4 )) to give rise to O 2 and water with the release of heat. H_2O_2(l)→H_2O(l)+1/2O_2(g) ΔG_298 K^o=-116.7 kJ mol^-1
 (4) Based on these considerations, one can anticipate that developing anodes with a high tolerance and low decomposition rate of H 2 O 2 are prerequisites for achieving high FE. Here, we develop a ZnGa 2 O 4 anode featuring dual active site for H 2 O 2 generation through WOR. At 2.3 V versus RHE, this ZnGa 2 O 4 shows its highest FE of ~82%. Significantly, by combining the in situ spectral evidence and theoretical calculations, it is identified that the generation of H 2 O 2 follows both the direct (OH - -mediated) and indirect (HCO 3 - -mediated) pathway at the ZnGa 2 O 4 anode. Theoretical studies indicate that bicarbonate species can bind with Ga-Ga dual sites and then be oxidized to percarbonate species. The O–O bond in peroxide species is stable on the surface of ZnGa 2 O 4 , which helps to maintain high FE and high H 2 O 2 concentration levels. Anode material characterizations The nanoflower-like ZnGa 2 O 4 was synthesized by the solvothermal method modified from a reported procedure [37] . The X-ray diffraction pattern of as-prepared sample is in accordance with that of spinel ZnGa 2 O 4 (PDF#38-1240) (Fig. 1a ), indicating a pure ZnGa 2 O 4 phase with high crystallinity. SEM image reveals the ZnGa 2 O 4 catalyst has a monodisperse microsphere with a uniform diameter of ~5 μm (Fig. 1b ). It is clearly shown a flower-like structure consisting of self-assembly nanosheets. From the transmission electron microscopy (TEM) images (Fig. 1c, d ), the nanosheets show irregular shape and clear lattice fringes were observed in the high-resolution TEM image (Fig. 1d and Figure S1 ), indicating the high crystallinity of the catalysts. The lattice fringes in Fig. 1d spaced 0.294 nm apart can be well assigned to the (220) facet of ZnGa 2 O 4 , and the lattice fringes spaced 0.25 nm apart (Figure S1c, d ) can be assigned to (311) facet. From the polycrystalline electron diffraction pattern (Fig. 1e ), it is found that the main diffraction spots correspond to the (440) facet (the secondary diffraction of the (220) facet) and the (311) facet. And in the selected area electron diffraction pattern (Figure S1b ), the diffraction spots corresponding to the (311) and (220) facets are clearly observed. Then using the scanning transmission electron microscopy electron energy loss spectroscopy (STEM-EELS) technique, as shown in Fig. 1f , a uniform elemental distribution is evidenced for the catalyst particles. Fig. 1: Morphological characterizations of ZnGa 2 O 4 . a X-ray diffraction pattern of the prepared ZnGa 2 O 4 . b SEM images of ZnGa 2 O 4 . c TEM image. d HRTEM image. e Polycrystalline electron diffraction pattern of ZnGa 2 O 4 . f Scanning transmission electron microscopy electron energy loss spectroscopy (STEM-EELS) of the ZnGa 2 O 4 . Full size image H 2 O 2 generation performance through selective water oxidation The ZnGa 2 O 4 anode was designed for anodic H 2 O 2 production (design principle can be found in Method part). As shown in Figure S2 , most ZnGa 2 O 4 particles are in single-particle dispersion on the anode surface rather than in agglomerates. For the electrochemical water oxidation reaction, as shown in Fig. 2a , the generation of H 2 O 2 is accompanied by the decomposition of H 2 O 2 on the anode surface (oxidation of H 2 O 2 to O 2 ) or in the bulk solution (Eq. ( 4 )). The H 2 O 2 generation performance evaluation is based on the accumulated H 2 O 2 concentration in the anolyte. From the LSV curves in Fig. 2b , the overpotential at 10 mA cm −2 of the ZnGa 2 O 4 anode was about 270 mV, suggesting a good water oxidation activity of the ZnGa 2 O 4 anode. Next, the FE of H 2 O 2 was evaluated in a potential range from 2.0 to 3.5 V versus RHE (details can be found in Table S2 ), and the corresponding current density was shown in Figure S3a . From Fig. 2c , the ZnGa 2 O 4 anode shows a FE as high as 38% at 2.0 V versus RHE. Significantly, the peak FE reaches 82% at 2.3 V versus RHE (overpotential of 540 mV), representing a high selectivity of ZnGa 2 O 4 towards H 2 O 2 formation. As shown in Fig. 2d , for example, maximum FE of 71% at 3.1 V versus RHE on BiVO 4 [38] , 76% at 3.2 V versus RHE on CaSnO 3 [24] , 81% at 3.1 V versus RHE on ZnO [25] , 28% at 3.17 V versus RHE on boron-doped diamond (BDD) [33] , 87% at 2.85 V versus RHE on BDD (B/D ratio = 0.012) [39] , 22% at 3.08 V versus RHE on Sb 2 O 3 [40] , 79% at 3.2 V versus RHE on Bi 2 WO 6 :5%Mo [7] , 8% at 2.9 V versus Ag/AgCl on C,N codoped-TiO 2 in an electrolyte of pH = 3 [35] . In comparison to these reported anodic materials that usually require overpotentials larger than 1000 mV to afford a high selectivity, the developed ZnGa 2 O 4 anode shows competitive FE at a low overpotential of 540 mV. Meanwhile, as shown in Table S3 , the current density of the ZnGa 2 O 4 anode is comparable to the reported performance at similar potentials. And the H 2 O-to-H 2 O 2 partial current density (Figure S3b ) is higher than that of previous oxide anodes [26] , [28] , [38] . At a potential equal to or higher than 2.3 V versus RHE, O 2 bubbles were observed on the anode surface, which is considered from the O 2 evolution reaction (OER). Fig. 2: Activity and stability of H 2 O 2 generation on ZnGa 2 O 4 anode. a Scheme of the electrochemical H 2 O 2 production on anodes through a water oxidation reaction. b LSV curves recorded in 2 M KHCO 3 before and after a stability test. The scan rate is 5 mV s −1 . c H 2 O 2 FE of the prepared ZnGa 2 O 4 anode at different potentials in 2 M KHCO 3 electrolyte (Error bars represent the standard deviation of three independent measurements). d The FE of typically reported anodes including ZnO [25] , boron-doped diamond (BDD) [33] , BDD (B/D ratio = 0.012) [39] BiVO 4 [38] , CaSnO 3 [24] , Bi 2 WO 6 :Mo [7] , and Sb 2 O 3 [26] for H 2 O 2 generation in bicarbonate/carbonate electrolyte for comparison. The orange star represents the thermodynamic potential of 2e-WOR. e The H 2 O 2 generation rate on the ZnGa 2 O 4 anode at different potentials. f The accumulated amount of H 2 O 2 in 60 min-electrolysis under different applied potentials, (50 mL electrolyte, electrode area = 0.5 cm 2 ). g The FE and generation rate of H 2 O 2 on ZnGa 2 O 4 anode with an applied bias of 2.3 V versus RHE in 700 minutes. The electrolyte was periodically replaced. Full size image The generation rate is another important parameter in evaluating the performance of catalysts. The H 2 O 2 generation rate of the ZnGa 2 O 4 anode at different potentials was measured (Fig. 2e ). The generation rate exceeds 10 μmol cm −2 min −1 at potentials higher than 2.7 V versus RHE. Such a high generation rate can meet the requirement of H 2 O 2 for many applications, including water disinfection (>1 mM) [41] , and Fenton reaction (>1 mM) [42] , [43] , [44] . In addition, it is found that higher concentrations of KHCO 3 lead to higher FE and generation rates for H 2 O 2 production (Figure S4 ). Then the accumulated amounts of H 2 O 2 in 60 minutes under different potentials (2.3, 2.5, and 2.7 V versus RHE) were recorded. The product formed on the anode would be desorbed into bulk solution and accumulates to high concentrations over time. As shown in Fig. 2f , the real-time concentration of H 2 O 2 increases almost linearly in 60 minutes, which indicates that the decomposition rate is not notable compared to the generation rate of H 2 O 2 . Finally, the cycle water oxidation tests were conducted at 2.3 V versus RHE (Figure S5 and Fig. 2g ). The electrolyte was periodically replaced to minimize the effect of changes in electrolyte composition. The H 2 O 2 FE was measured for each test cycle (Fig. 2g ), and a FE of ~78% was maintained after 700 min of continuous electrolysis. It also reveals that the generation rate decreased from 6.27 to 5.95 μmol cm −2 min −1 after 700 minutes of stability test. The LSV curve (Fig. 2b ) was also recorded after the stability test and no apparent changes were observed in the comparison. The flower-like morphology of the ZnGa 2 O 4 catalyst on the anode surface was retained after the stability test (Figure S6 ). By comparing the high-resolution X-ray photoelectron spectroscopy spectra of Zn 2 p and Ga 3 d obtained before and after the stability test, it can be inferred that the valence state of metal ions in this spinel structure is stable after the electrolysis test (Figure S7 ). The nearly unchanged LSV curves before and after the stability test, the slightly decreased FE after the 700-min electrolysis, and the unchanged morphology indicate the excellent durability of ZnGa 2 O 4 catalyst under water oxidation conditions. According to recent progress, anodic H 2 O 2 production was also achieved in carbonate-based electrolytes [45] , [46] , [47] . Here, the H 2 O 2 production performance of ZnGa 2 O 4 anode in 2 M K 2 CO 3 solution was then investigated (Figure S8 ). The ZnGa 2 O 4 can afford a much higher current density in 2 M K 2 CO 3 (Figure S8a ) than in 2 M KHCO 3 (Fig. 2b ). The highest FE reaches 77%, but the corresponding potential is as high as 2.9 V versus RHE (Figure S8b ). Figure S8c shows that the highest H 2 O 2 generation rate of ~69 μmol cm −2 min −1 was achieved at 3.1 V versus RHE, which is much higher than that in 2 M KHCO 3 electrolyte (21 μmol cm −2 min −1 at 3.1 V versus RHE). Next, at 2.9 V versus RHE, H 2 O 2 concentration reaches 54 mM after 150 minutes (Figure S8d ). Decomposition of H 2 O 2 during electrolysis The real-time concentration of H 2 O 2 in the anolyte over several hours is essential for realistic applications. Herein, the H 2 O 2 concentration in 300 minutes was recorded under potentials of 2.3, 2.5, and 2.7 V versus RHE (Fig. 3a ), and the corresponding current density can be found in Figure S9 . 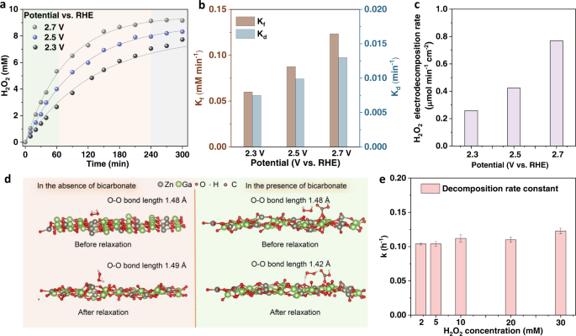Fig. 3: The accumulation and decomposition of H2O2. aThe real-time H2O2concentration as a function of time at 2.3, 2.5, and 2.7 V versus RHE. (60 mL electrolyte, electrode area = 0.5 cm2). The solid lines are the fitting curves.bThe formation rate constant and decomposition rate constant of H2O2on ZnGa2O4anode at different potentials.cElectrodecomposition rate of H2O2on ZnGa2O4anode at different potentials in 2 M KHCO3.dStructure of H2O2-ZnGa2O4before and after relaxation in the absence of bicarbonate (left) and the presence of bicarbonate (right).eSelf-decomposition rate constants of H2O2with different initial concentrations in 2 M KHCO3solution. Error bars represent the standard deviation of three independent measurements. Figure 3a reveals that the H 2 O 2 concentration curves deviate obviously from the linear growth trend after 60 minutes-electrolysis and then reach a plateau after 240 min-electrolysis. The declining growth rate should be related to the decomposition of high concentrations of H 2 O 2 in the electrolyte. At constant potential, the formation rate of H 2 O 2 can be described as zero-order kinetics, and the decomposition of H 2 O 2 follows the first-order kinetics related to the H 2 O 2 concentration ([H 2 O 2 ]) [48] , [49] , [50] . The formation rate (r f ) equals to K f ( K f : formation rate constant); the decomposition rate ( r d ) equals K d [H 2 O 2 ], ( K d : decomposition rate constant). Thus, the real-time H 2 O 2 concentration can be expressed as: 
    [H_2O_2]=(K_f/K_d)[1-exp(-K_dt)]. (5) Fig. 3: The accumulation and decomposition of H 2 O 2 . a The real-time H 2 O 2 concentration as a function of time at 2.3, 2.5, and 2.7 V versus RHE. (60 mL electrolyte, electrode area = 0.5 cm 2 ). The solid lines are the fitting curves. b The formation rate constant and decomposition rate constant of H 2 O 2 on ZnGa 2 O 4 anode at different potentials. c Electrodecomposition rate of H 2 O 2 on ZnGa 2 O 4 anode at different potentials in 2 M KHCO 3 . d Structure of H 2 O 2 -ZnGa 2 O 4 before and after relaxation in the absence of bicarbonate (left) and the presence of bicarbonate (right). e Self-decomposition rate constants of H 2 O 2 with different initial concentrations in 2 M KHCO 3 solution. 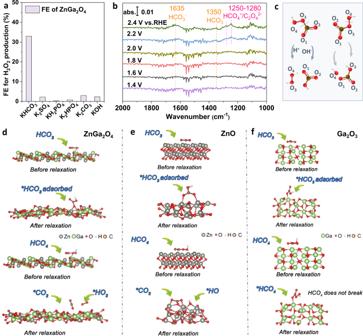Fig. 4: The bicarbonate species-mediated reaction pathway. aThe H2O2FE of ZnGa2O4anode in different electrolytes (0.5 M) at a constant current of 8 mA cm−2.bIn situ Fourier transform infrared spectra of ZnGa2O4at different potentials in 2 M KHCO3.cTwo possible decomposition ways of HCO4on the catalyst surface. Models ofdHCO3-ZnGa2O4and HCO4-ZnGa2O4at (311) facet,eHCO3-ZnO and HCO4-ZnO,fHCO3-Ga2O3and HCO4-Ga2O3before and after structure relaxation. 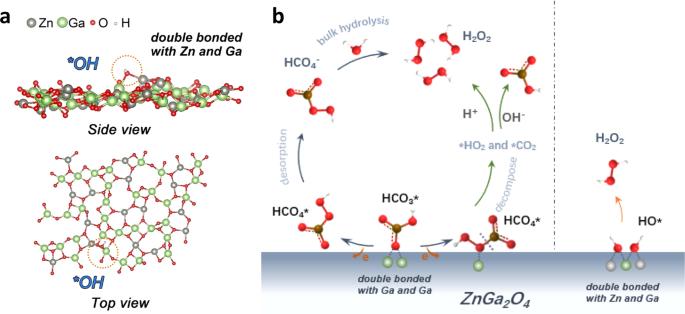Fig. 5: Proposed reaction pathways of water oxidation to H2O2. aSide view and top view of adsorption of *OH on ZnGa2O4.bScheme illustration of the proposed direct and indirect pathways toward H2O2generation on the ZnGa2O4surface. Error bars represent the standard deviation of three independent measurements. Full size image Then according to the fitting results (Fig. 3a ), the K f under 2.3, 2.5 and 2.7 V versus RHE were calculated to be 0.06, 0.088, and 0.123 mM min −1 , respectively. The corresponding K d under 2.3, 2.5, and 2.7 V versus RHE was calculated to be 0.008, 0.01, and 0.013 min −1 (Fig. 3b ). These results indicate that the formation and decomposition rate constants (i.e., K f , K d ) are increased at higher potentials. In consequence, the decomposition rate ( r d ) increases at more positive potentials. As shown in Figure S10 , the apparent generation rates of H 2 O 2 in 300 min-electrolysis gradually decrease over time because of H 2 O 2 decomposition, which can be caused by the anode materials (electrodecomposition and chemical decomposition on anode surface), H 2 O 2 disproportionation in the electrolyte, and the changes of the anolyte composition [46] during electrolysis. To evaluate the electrodecomposition of H 2 O 2 on the ZnGa 2 O 4 anode, a current integration method (details can be found in the Method) was used [51] . As shown in Figure S11 , at 2.3 and 2.5 V versus RHE, there is no significant increase in the current when adding 10 mM H 2 O 2 to the electrolyte. The corresponding electrodecomposition rates are calculated to be 0.26, 0.42, and 0.77 μmol cm −2 min −1 at 2.3, 2.5, and 2.7 V versus RHE (in Fig. 3c ), suggesting the higher electrodecomposition rates of H 2 O 2 at more positive potentials. Therefore, the ZnGa 2 O 4 anode affording high FE at a low potential can help to suppress the electrodecomposition of H 2 O 2 . Meanwhile, it has been reported that catalysts themselves can also induce the chemical decomposition of H 2 O 2 [52] . Figure S12 shows a negligible difference in H 2 O 2 stability between the control experiments, indicating that ZnGa 2 O 4 would not decompose the generated H 2 O 2 . The influence of bicarbonate on H 2 O 2 stability was then also explored, as adsorbed bicarbonate species have been reported to decompose the formed H 2 O 2 [53] . The stability of the peroxy bond of H 2 O 2 on ZnGa 2 O 4 surface with and without bicarbonate anions was also examined by theoretical calculations. The bond length of O-O almost maintains its initial value after structure relaxation (Fig. 3d left ). This indicates that the peroxy bond is less likely to decompose on the surface of ZnGa 2 O 4 . Similarly, on the surface of ZnGa 2 O 4 with bicarbonate adsorbed, the bond length of O-O does not increase and the structure of H 2 O 2 does not change greatly (Fig. 3d right). As a result, two hydrogen bonds are formed with one linked to the bicarbonate and another one linked to the oxygen atom from the ZnGa 2 O 4 substrate, suggesting the H 2 O 2 is less likely to decompose on the surface of ZnGa 2 O 4 with adsorbed bicarbonate. In addition to the decomposition on the anode, H 2 O 2 would undergo disproportionation (Eq. ( 4 )) in weak alkaline solutions or with the presence of metal impurities (usually transition-metal ions) [54] . Figure S13 records the remaining ratio of H 2 O 2 with different initial concentrations ([H 2 O 2 ] 0 ) as a function of time. More than 60% of H 2 O 2 self-decomposed after 360 minutes at room temperature when [H 2 O 2 ] 0 is in the range of 2–30 mM, indicating that the disproportionation can cause severe loss of H 2 O 2 . Similarly, a decrease of 19% in H 2 O 2 concentration (from 1.1 to 0.89 mM) at an open circuit after 150 minutes was reported by Pangotra et al. [46] . The linear fitting curves in Figure S13 indicate that the disproportionation of H 2 O 2 in 2 M KHCO 3 solution is a zero-order reaction. Accordingly, the decomposition rate constants are determined to be 0.10 ~ 0.12 h −1 (Fig. 3e , details can be found in Figure S13 ). At last, the changes in conductivity and pH of anolyte were explored. In Figure S14 , a decrease in conductivity (~ 3%) and an increase in pH (from 8.31 to 8.68) were recorded at 2.3 V versus RHE during the 300 minutes-electrolysis. It is considered that such slight changes in the electrolyte were not the main factors for the declined H 2 O 2 generation rate. Therefore, for the anodic H 2 O 2 production in the absence of a stabilizer, an integrated effect of H 2 O 2 decomposition (in the bulk solution and at the anode surface) as well as the changes in electrolytes leads to the concentration plateau during continuous electrolysis. For the ZnGa 2 O 4 anode, the above evidence reveals that disproportionation instead of the electrode composition is mainly responsible for the H 2 O 2 concentration plateau. Proposed reaction pathways Then the reaction pathway is further investigated. First, the ZnGa 2 O 4 anode was tested in other electrolytes including K 2 SO 4 , K 2 HPO 4 , KH 2 PO 4, K 2 CO 3, and KOH to study the effect of electrolyte composition on H 2 O 2 generation. Considering that the above electrolytes have different oxidation potentials, the FE of H 2 O 2 in different electrolytes was also tested at a constant current density (8 mA cm −2 ) by the chronopotentiometry method. The results are shown in Fig. 4a and Figure S15 , it is found that the FE of H 2 O 2 in 0.5 M KHCO 3 , 0.5 M K 2 SO 4 , 0.5 M KH 2 PO 4 , 0.5 M K 2 HPO 4 , 0.5 M K 2 CO 3 , and 0.5 M KOH are 32.5%, 2%, 0.3%, 0.8%, 3%, 2.3%, respectively. These observations indicate that HCO 3 − anions play an indispensable role in tailoring the selectivity of water oxidative reaction on the ZnGa 2 O 4 anode. At potentials above 1.9 V versus RHE, it is accepted that the reaction mainly follows a direct water oxidation pathway (H 2 O/OH − to H 2 O 2 ) in K 2 SO 4 , K 2 HPO 4 , and KH 2 PO 4 . However, in the presence of HCO 3 - , competing reactions involving the oxidation of HCO 3 − may occur on the anode surface ( E (HCO 4 − /HCO 3 − ) = 1.8 ± 0.1 V versus NHE) [29] . To gain insight into the evolution of HCO 3 − on the anode, experimental and theoretical investigations were conducted to explore the adsorption properties of these species. Fig. 4: The bicarbonate species-mediated reaction pathway. a The H 2 O 2 FE of ZnGa 2 O 4 anode in different electrolytes (0.5 M) at a constant current of 8 mA cm −2 . b In situ Fourier transform infrared spectra of ZnGa 2 O 4 at different potentials in 2 M KHCO 3 . c Two possible decomposition ways of HCO 4 on the catalyst surface. Models of d HCO 3 -ZnGa 2 O 4 and HCO 4 -ZnGa 2 O 4 at (311) facet, e HCO 3 -ZnO and HCO 4 -ZnO, f HCO 3 -Ga 2 O 3 and HCO 4 -Ga 2 O 3 before and after structure relaxation. Full size image The \({{HCO}}_{3}^{-}\) -mediated water oxidation pathway The effect of bicarbonate on boosting FE of water oxidation towards H 2 O 2 has ever been observed by our group [8] and others [29] , [55] . However, this proposed reaction pathway needs more solid evidence and in-depth investigation. Here, in situ attenuated total reflectance Fourier transform infrared spectroscopy (ATR-FTIR) technique was used to probe the reaction intermediates. A schematic representation of the electrochemical cell used for ATR-FTIR test can be found in Figure S16 . In Fig. 4b , above 1.8 V versus RHE, the FTIR peaks at 1635 cm −1 and 1350 cm −1 are related to the symmetric C-O stretch of the adsorbed HCO 3 − [56] . When the applied potential increased to 2.2 V versus RHE, new FTIR bands were observed, and the intensity of bands become stronger at 2.4 V versus RHE. Specifically, the FTIR bands at 1286 cm −1 (valence C=O sym.) and 1265 cm −1 (C=O) can be matched to the symmetric C=O stretch of HCO 4 − /C 2 O 6 2- [57] , [58] , indicating the formation of percarbonate species on the surface of ZnGa 2 O 4 . Therefore, the in situ spectral identifications prove the indirect reaction pathway for H 2 O 2 generation via the transformation of bicarbonate to percarbonate species. Next, models with \({{{{{{\rm{HCO}}}}}}}_{3}^{-}\) or \({{{{{{\rm{HCO}}}}}}}_{4}^{-}\) on the anode surface are constructed to explore the adsorption properties of bicarbonate species. The oxygen atoms of HCO 4 - are labeled for convenient discussion (Fig. 4c ). As shown in Fig. 4d , after structure relaxation, the HCO 3 − could be adsorbed stably on the (311) facet of ZnGa 2 O 4 by forming a bridged adsorption configuration (the O 1 atom of *HCO 3 binding with two Ga atoms). The adsorption energy is calculated to be −1.9 eV according to the following equation: 
    E_ad=E_tot-E_sub-E_inter. (6) Where E ad is the adsorption energy, E tot is the total energy of the system, E sub is the energy of the substrate and E inter is the energy of HCO 3 − intermediate. The negative value of E ad confirms that the HCO 3 − adsorption on the (311) facet of ZnGa 2 O 4 is favorable. As revealed by the in situ ATR-FTIR spectra, the adsorbed bicarbonate (*HCO 3 ) can be oxidized to percarbonate species (*HCO 4 ) on the surface of ZnGa 2 O 4 . Meanwhile, we also used theoretical calculations to study the energy change of the system (Theoretical calculations can be found in Method). In the theoretical calculations, (311), (220) and ( \(\bar{1}\) 12) facets were all considered. On (311) facet, the energy of the HCO 4 -ZnGa 2 O 4 system decreases by 1.82 eV compared to that of HCO 3 -ZnGa 2 O 4 at 2.3 V versus RHE at 298 K (Fig. 4d ). The energy decreases by 0.16 eV on the (220) facet and decreases by 0.39 eV on the ( \(\bar{1}\) 12) facet at 2.3 V versus RHE at 298 K (Figure S17 , S18 , the energy changes are summarized in Table S4 ). These results indicate that the conversion of *HCO 3 to *HCO 4 on (311), (220), and ( \(\bar{1}\) 12) facets of ZnGa 2 O 4 is thermodynamically favorable. It is inferred that the conversion of *HCO 3 to *HCO 4 originates from the special dual adsorption sites of *HCO 3 on ZnGa 2 O 4 . Then to gain insight into the HCO 3 − mediated pathway on the ZnGa 2 O 4 anode, the adsorption properties of bicarbonate and percarbonate on ZnO and Ga 2 O 3 were also investigated for comparison. For the model of ZnO-*HCO 3 , two oxygen atoms (O 1 and O 2 ) of *HCO 3 adsorb with two Zn atoms (Fig. 4e top) separately, suggesting ZnO is favorable for *HCO 3 adsorption. In the case of Ga 2 O 3 , the *HCO 3 adsorbs on the surface of Ga 2 O 3 by forming a single adsorption site of Ga (Fig. 4f ). The formed HCO 4 - species on the anode surface can be desorbed into the bulk electrolyte, followed by a hydrolysis process to give H 2 O 2 [55] . Alternatively, as a highly reactive species, the HCO 4 - may also undergo decomposition on the anode surface. According to DFT results, in the models of HCO 4 -ZnGa 2 O 4 (Fig. 4d bottom, S17b, and S18b), the *HCO 4 will decompose into *CO 2 and *O 2 H by cleaving the -C-O 3 - bond after structure relaxation. Then the *CO 2 will dissolve into the solution and form HCO 3 - by combing OH - anions, while *O 2 H, containing the -O-O- bond, would transform to H 2 O 2 . In such transformation, the peroxy bond keeps intact, representing one of the advantages of the ZnGaO 4 anode. However, on the surface of ZnO, the *HCO 4 would decompose to *CO 3 and *OH by breaking the –O 3 –O 4 - bond (Fig. 4e ). This may be caused by the strong interaction between the O atoms of percarbonates and the Zn sites. This decomposition may also be affected by the initial adsorption states. As shown in Fig. 4e , the O 1 and O 2 atoms of the *HCO 3 form two Zn-O bonds with the ZnO substrate. This is different from the situation on ZnGa 2 O 4 , where two Ga are bonded with only one oxygen atom of * HCO 3 . Although both cases are dual-site adsorption, the –C–O 3 - bond of *HCO 4 is less likely to be cleaved on the ZnO model. Instead, the *HCO 4 will decompose to *CO 3 and *OH by breaking the peroxy bond on ZnO. Then three O atoms of the *CO 3 are bonded with Zn atoms as shown in Fig. 4e . In the case of Ga 2 O 3 , the *HCO 4 is just stably adsorbed on the anode surface (Fig. 4f ), where the O 1 or O 2 atom of *HCO 4 is bonded with a Ga site. Such adsorption configuration avoids the decomposition of *HCO 4 . The OH - -mediated water oxidation pathway The generation of H 2 O 2 in electrolytes without bicarbonate (Fig. 4a ) indicates the direct water oxidation reaction on ZnGa 2 O 4 anode. Prior studies have proposed that the adsorption energy of *OH (ΔG *OH ) on the surface of the catalyst determines the selectivity of WOR [38] , [59] . Small ΔG *OH often causes the evolution of O 2 while large ΔG *OH leads to the formation of ·OH radicals. To produce H 2 O 2 , a suitable ΔG *OH should be smaller than 2.4 eV and larger than 1.6 eV. According to DFT results, after relaxation, it is discovered that *OH can adsorb on the surface of ZnGa 2 O 4 with an energy of 1.63 eV, which is within the optimum range for H 2 O 2 generation. Interestingly, the O atom in *OH is bonded with Zn and Ga atoms (Fig. 5a ). The bond length of Zn-O is 1.97 Å, and the bond length of Ga-O is 2.04 Å. The similar bond length confirms the formation of a dual-site (Zn-Ga) adsorption configuration. As a result, the water oxidation to H 2 O 2 molecules is reasonably inferred at this Zn-Ga region with a dual-adsorption site. A detailed energy diagram of the reaction steps involved in the OH - -mediated water oxidation pathway was shown in Figure S19 . In addition, as shown in Figure S20 , the distinct advantage of the HCO 3 -mediated pathway in promoting anodic H 2 O 2 generation was also observed on some other anodes including F-doped tin oxide (FTO), FTO/WO 3 , and Toray TGP-H-060 carbon fiber paper (CFP). For example, the H 2 O 2 FE of FTO, FTO/WO 3 , and CFP are 5%, 13%, and 9% in 0.5 M KHCO 3 . However, the H 2 O 2 FE is below 0.5% for all three anodes in 0.5 M KOH. Fig. 5: Proposed reaction pathways of water oxidation to H 2 O 2 . a Side view and top view of adsorption of *OH on ZnGa 2 O 4 . b Scheme illustration of the proposed direct and indirect pathways toward H 2 O 2 generation on the ZnGa 2 O 4 surface. Full size image Overall, on this ZnGa 2 O 4 anode, H 2 O 2 can be generated through either the HCO 3 - -mediated reaction pathway or the OH - -mediated reaction pathway (Fig. 5b ). The former plays a critical role in boosting H 2 O 2 FE. Meanwhile, DFT results indicate that the conversion of *HCO 3 to *HCO 4 relies on the dual-adsorption site (Ga-Ga) of ZnGa 2 O 4 . Furthermore, percarbonate species may undergo decomposition on the electrode surface, giving rise to *CO 2 and*HO 2 by breaking the –C–O– bond or *CO 3 and *HO by breaking the -–O–O– bond (Fig. 5b ). The latter causes a decrease in FE because the crucial intermediate HCO 4 - was eliminated. The theoretical studies indicate that the high H 2 O 2 FE of ZnGa 2 O 4 is related to the conversion of *HCO 3 to *HCO 4 at the dual-site, and to the intact peroxides on the surface of ZnGa 2 O 4 . Therefore, the FE is not only determined by the reaction selectivity but also influenced by the stability of the peroxy bond on the anode surface. Next, the real-time H 2 O 2 concentration was recorded when applying a potential of 2.7 V versus RHE to the anode (Figure S21 ). It is found that the H 2 O 2 concentration increases linearly in the first 60 minutes and then the growth slows down. The H 2 O 2 concentration reaches a plateau after 200 minutes owing to H 2 O 2 disproportionation and electrodecomposition. After 300 min-electrolysis, the H 2 O 2 concentration reaches ~22 mM. It is worth noting that such a concentration has met the requirement of applications such as the Fenton reaction (> 1 mM) [42] , [60] , [61] , water disinfection (>1 mM) [41] . In conclusion, a highly selective ZnGa 2 O 4 anode was developed for H 2 O 2 production by oxidizing water, delivering a high FE of 82% at a low overpotential of 540 mV, along with good stability. In this case, it is revealed that the H 2 O 2 concentration plateau during continuous electrolysis up to 5 h is largely realted to homogeneous decomposition (disproportionation) instead of electro decomposition. Based on our experimental observations and the theoretical calculations, the H 2 O 2 is formed on ZnGa 2 O 4 through both the indirect and direct reaction routes. More importantly, the indirect route, mediated by the HCO 3 - /HCO 4 - , is the critical route for H 2 O 2 production. ZnGa 2 O 4 favors the adsorption of HCO 3 - at the dual Ga-Ga sites. The conversion of *HCO 3 to *HCO 4 on ZnGa 2 O 4 is confirmed by the in situ ATR-FTIR spectra and the energy change in DFT results. Significantly, adsorbed *HCO 4 was found to decompose into *CO 2 and *O 2 H, and the latter would transform into H 2 O 2 . Additionally, the peroxy bond in H 2 O 2 and HCO 4 - is stable on the ZnGa 2 O 4 surface with and without HCO 3 - anions. As well-known, the anodic H 2 O 2 generation performance can be affected by the supporting electrolyte [27] , [45] , [46] , [62] . For this ZnGa 2 O 4 anode, given the high FE in bicarbonate as well as the large current density in carbonate solution for anodic H 2 O 2 generation, further study can be focused on optimizing the composition of electrolytes further to improve the FE of ZnGa 2 O 4 for H 2 O 2 production and to elucidate the reaction mechanism behind it. Preparation of catalyst and electrodes The ZnGa 2 O 4 anode was designed for anodic H 2 O 2 formation because of the following reasons. Firstly, it is important to avoid the decomposition effect of the catalyst itself on H 2 O 2 . Thus, some metal cations cannot be chosen. For example, catalysts that can decompose H 2 O 2 into O 2 [29] , [52] (MnO 2 and CoO) or catalysts containing Fe or Mn elements that can activate H 2 O 2 into hydroxide radicals [63] should be excluded. Secondly, to improve the selectivity of H 2 O 2 , competitive reactions such as oxygen evolution and the formation of hydroxyl radicals should be suppressed on the anode surface. The strength of oxygen chemisorption on transition metal (TM) ions should be taken into consideration when designing the catalysts for electrochemical water oxidation. Numerous efforts have revealed that the oxygen chemisorption strength on a metal surface is related to its electronic structure, i.e. the position of the metal’s d-band center relative to its Fermi level [64] , [65] , [66] , [67] . Those TM atoms such as Co, Ni, Fe, Mn featuring suitable chemisorption of oxygen on the catalyst surface were excluded because *OH can be easily dissociated into *O and finish the 4e-water oxidation pathway. Thirdly, according to the previous researches, the most reported anode materials for H 2 O 2 production are those TM oxides containing cationic ions with closed electronic shell configurations, such as W 6+ (5d 0 ), Bi 3+ (6s 2 ), Zn 2+ (3d 10 ), Sn 4+ (4d 10 ). It is possible that the dominance of this configuration is related to the inert oxygen evolution activity of these metal oxides. Therefore, we designed ZnGa 2 O 4 anode in which Zn and Ga have closed electronic shell configurations to investigate the anodic H 2 O 2 generation performance. Besides, the good chemical stability of ZnGa 2 O 4 in oxidative condition is also beneficial to 2e-WOR, which has been demonstrated in previous studies [37] , [68] , [69] , [70] . The ZnGa 2 O 4 microsphere was prepared according to a previous report with minor modifications [37] . Gallium nitrate hydrate and zinc acetate were dissolved in pure water (10 mL) with a molar ratio of 2:1. To obtain the flower-like structure consisting of nanosheets, the concentration of zinc precursor was optimized to 25 mM. Then 5 mL of ethylenediamine was added to the above solution and stirred at room temperature for 20 min. Next, the mixture was transferred to a 25 mL autoclave and heated at 200 °C for 16 h. After cooling down to room temperature, the sample was obtained by centrifugation and washed with deionized water and ethanol several times in sequence. Then the sample was dried at 60 °C overnight. After cleaning with ethanol three times, the carbon fiber cloth (Taiwan Tanneng, WOS1009) was dried at room temperature. Next, 300 mg ZnGa 2 O 4 catalyst and 30 mg polytetrafluoroethylene were dispersed in 10 mL ethanol, followed by a sonication treatment for 20 min to form a highly dispersed mixture. Then the cleaned CC was placed on a hot plate (150 °C), and the ZnGa 2 O 4 catalyst mixture was painted onto the CC by brushing, followed by a heat treatment at 350 °C for 30 min in Argon flow. The loading amount of ZnGa 2 O 4 was about 20 mg cm −2 . Characterizations Phase identification was conducted on a Rigaku SmartLab X-ray diffractometer with Cu Kα irradiation (λ = 1.5406 Å) operation at 40 kV and 40 mA. X-Ray photoelectron spectroscopy (XPS) characterizations of samples before and after electrolysis or Fenton reaction were obtained on a Thermo ESCALAB 250Xi spectrometer equipped with an anode of Al Kα radiation (1486.6 eV) X-ray sources. The obtained XPS data were calibrated by the C1 s position (284.8 eV) before the data process. For the quantification of the formed H 2 O 2 from anode under different biases, the concentration of H 2 O 2 was quantified based on the spectrophotometric determination of I 3 − [71] . Firstly, solutions A and B were prepared for the quantification of H 2 O 2 by I 3 − method. To prepare solution A, 33 g KI, 1.4 g KOH, and 0.1 g (NH 4 ) 6 Mo 7 O 24 ·4H 2 O were dissolved in 500 mL distilled water. 10 g potassium hydrogen phthalate was dissolved in 500 mL distilled water as solution B. Solution A should be kept in the dark to inhibit the oxidation of I − . The pH of the sample solution was adjusted to 7 before the test. Then the sample solution, solutions A and B were mixed in equal volumes. After 5 min, the UV absorption spectrum of the mixture solution was recorded on Cary Series UV-Vis Spectrometer (Agilent Technologies). The accumulated concentration of H 2 O 2 in the anolyte was quantified, based on which the faradaic efficiency and production rate are calculated. Scanning electron microscopy (SEM) characterizations were performed on an FEI Quanta 400 microscope. The transmission electron microscopy (TEM) and high-resolution TEM were conducted on a Philips Tecnai F20 instrument and a CM-120 microscope (Philips, 120 kV). ATR-FTIR measurement For the attenuated total reflectance Fourier transform infrared spectroscopy (ATR-FTIR) test, a single Si crystal (diameter: 20 mm) was used as an ATR crystal. A high-sensitivity mercury calcium telluride (MCT) detector and optical path accessories with high luminous flux were required to detect the adsorption vibration signals. The spectral signal was collected by a Fourier transform infrared spectroscopy (FTIR, Thermo Scientific Nicolet iS50). A rough Au film with good conductivity was deposited onto the ATR crystal to enhance the infrared absorption by means of the local electric field of the surface plasmon. In the three-electrode system, Pt wire was used as the counter electrode, and catalyst film on the Si crystal (coated with Au film) acts as the working electrode connected to the external circuit through a copper foil. A schematic representation of the in situ electrochemical cell for the ATR-FTIR test is shown in Figure S16 . The data recorded at open circuit potential was used as the background. All the spectra were recorded in the range of 4000 ~900 cm −1 with a resolution of 4 cm –1 and averaged with 32 scans. Electrochemical measurements Electrochemical experiments in a three-electrode set-up were performed on a CHI 760E electrochemical station (CH Instruments, Inc., Shanghai). Potentials set against Ag/AgCl were converted to the RHE scale according to E RHE = E Ag/AgCl + 0.197 + 0.059 × pH, and the pH values of electrolytes value were tested by a pH meter (FE28, Mettler Toledo, Switzerland). The conductivity of the electrolyte was measured with a conductivity meter (DDS-307A, Shanghai INESAScientific Instrument Co., Ltd., China). The water oxidation performance of anodes was evaluated in a two-compartment cell divided by a Nafion 117 membrane (DuPond Co.). A Pt foil and a Ag/AgCl electrode (in a Luggin capillary) were used as the counter, and reference electrode, respectively. The electrochemical tests were performed without iR-compensation. Both of the compartments of the H-cell were full with 2 M KHCO 3 solution, and the electrolyte was stirred at a rate of 600 r.p.m. during the electrochemical test. After passing a particular amount of coulombs (depending on the applied potentials), 0.5 mL anolyte was taken out and the H 2 O 2 concentration in it was quantified by the I 3 - method. For the cyclic electrochemical tests, the electrolyte was periodically replaced. The overpotential is calculated as follows: 
    Overpotential=E_applied-E_thermodynamic of2e-WOR=E_appliedversus RHE-1.76V versus RHE. (7) E applied is the potential applied to the anode during tests. Evaluation on the electrodecomposition of H 2 O 2 on the ZnGa 2 O 4 anode The standardized method for measuring the electrodecomposition (ED) of H 2 O 2 on anodes during anodic H 2 O 2 production has yet to be well established. Here, a current integration method, i.e. to compare the faradaic charge with and without H 2 O 2 (known concentration) at the same applied potential, was used to evaluate the electrodecomposition of H 2 O 2 on ZnGa 2 O 4 anode [51] . Specifically, chronoamperometric courses of ZnGa 2 O 4 anode at potentials (2.3, 2.5, 2.7 V vs. RHE) in 2 M KHCO 3 solution with and without H 2 O 2 (10 mM) were recorded (Figure S10 ). Then the total faradaic charge passed in solution with and without H 2 O 2 addition was compared, and the difference between the two tests is assumed to be the charge corresponding to the oxidation of H 2 O 2 . Taking the analysis at 2.3 V vs. RHE as an example, the calculation details are shown below. ∫_0s^300sI_KHCO3 without H2O2 tdt=Q_KHCO3 without H2O2
 (8) 
    ∫_0s^300sI_KHCO3 with H2O2tdt=Q_KHCO3 with H2O2
 (9) 
    FE_ED,current intergration=Q_KHCO3 with H2O2 - Q_KHCO3 without H2O2/Q_KHCO3 with H2O2
 (10) 
    =3.732 C-3.578 C/3.732 C=0.041
 
    H_2O_2_Electrodecomposition	=H_2O_2_Accumulated×FE_ED,current intergration
     	=6.27 μmol min^-1cm^-2× 0.041 
     	=0.26 μmol min^-1cm^-2
 (11) \({{H}_{2}{O}_{2}}_{{{{{{\rm{Accumulated}}}}}}}\) means the measured H 2 O 2 generation rate (6.27 μmol cm −2 min −1 at 2.3 V vs. RHE in Fig. 2e ). \({{FE}}_{{ED},{current\; intergration}}\) at 2.5 and 2.7 V vs. RHE are 0.047 and 0.059. The electro decomposition rate of H 2 O 2 at 2.5 and 2.7 V vs. RHE in 2 M KHCO 3 are calculated to be 0.42 and 0.77 μmol cm -2 min -1 . It should be noted that this method provides an overestimation of the role of H 2 O 2 electro decomposition because the concentration of H 2 O 2 added during the tests (10 mM) is higher than the concentration plateau observed in Fig. 3a . Such approximate evaluation of the electro decomposition of H 2 O 2 can help to identify the main factors causing the decomposition of H 2 O 2 . Theoretical calculations The mechanism for H 2 O 2 generation is studied by using VASP computational package [7] . Projector-augmented-wave method with the Perdew–Burke–Ernzerhof GGA functional was used [72] . The electronic convergence limit was set to be 1 × 10 −5 eV [73] . Optimization of atomic coordinates was considered to be converged when Hellmann–Feynman force was smaller than 1× 10 −2 eV Å −1 . The established slab of ZnGa 2 O 4 is (311) facets with Zn and Ga atoms termination. Besides, the established slab of ZnO is (200) facets with Zn atoms termination. The established Ga 2 O 3 slab is (020) facets with Ga atoms termination. Intermediate including *OH, *HCO 3 and *HCO 4 is separately placed on the top of the slab surface. The vacuum region is about 10 Å in height. The surface termination for the DFT studies was determined based on the XRD pattern, the polycrystalline diffraction patterns, and the HRTEM images. We first choose the (311) facet because it is the strongest diffraction peak in the XRD pattern of the ZnGa 2 O 4 catalyst, which indicates that (311) facets should widely exist in the crystals. This approach has been used in previous reports on electrocatalysts with a cubic spinel structure, where the theoretical calculations are based on the observed main peaks in the XRD pattern [74] , [75] , [76] . For example, a previous report (Nat. Catal. 2022, 5, 109-118) studied the Co 2 MnO 4 (space group Fd \(\bar{3}\) m, a = 8.0866 Å ), the DFT calculation was conducted based on the (311) surface (the dominant peak in the PXRD) [75] . Since (311) and (220) facets are also observed in the HRTEM images (Fig. 1d and S1c, d), it can be concluded that (220) and (311) facets widely exist in the prepared ZnGa 2 O 4 catalyst. It is necessary to investigate the adsorption of reaction intermediates on both (311) and (220) facets. Finally, in the selected area electron diffraction pattern (Figure S1b ), considering that the zone axis perpendicular to (311) and (220) facets is [ \(\bar{1}\) 12], ( \(\bar{1}\) 12) facet is also considered in our calculations. Next, the conversion of *HCO 3 to *HCO 4 on these three facets was investigated. Here, by using the computational hydrogen electrode method to identify the conversion of bicarbonate to percarbonate is thermodynamically favorable or not. The influence of applied potential is considered via computational hydrogen electrode (CHE) method [77] , [78] . In this method, at standard condition, chemical potential of proton and electron is equals to that of a half of hydrogen gas (μ(H + + e - ) = 1/2 μ(H 2 )). The potential of the electrons is eU, where e is the elementary charge and U is the potential applied to the electrode. The catalytic process on the surface is investigated by calculating the energy of intermediates during the process. The transfer of *HCO 3 to *HCO 4 should involve the following step: 
    ∗HCO_3^-+∗OH^-=∗HCO_4^-+H^++2e. (12) Based on the above step, the computational change of energy of the intermediates adsorbed on the surface can be calculated according to the following method: 
    E=E_*HCO4-E_*HCO3+0.5E_H2-E_OH-2eU. (13) Where E *HCO4 , E *HCO3 , E H2 , and E OH is the adsorption energy of HCO 3 , HCO 4 , H 2 , and OH, and U is the applied potential. The Gibbs free energy changes of intermediates were calculated with zero-point energy, and entropy correction using the equation bellows: 
    At  T=0K, G=E+ZPE-TS. (14) Where, ZPE, T, and S correspond to zero-point energy, temperature, and entropy, respectively. In the case of the (311) facet, the E *HCO4− E *HCO3 is calculated to be −1.00 eV, E H is −3.39 eV, E OH is −7.34 eV, U is 2.3 V. Therefore, ∆E is calculated to be −1.65 eV (E *HCO4− E *HCO3 + E H - E OH - 2eU). The ZPE for HCO 3 is 0.66 eV; ZPE for HCO 4 is 0.80 eV; ZPE for H is 0.16 eV; ZPE for OH is 0.33 eV; ∆ZPE is −0.03 eV (0.80 eV–0.66 eV + 0.16 eV–0.33 eV = 0.03 eV). At 298 K, TS for HCO 3 is 0.05 eV; TS for HCO 4 is 0.14 eV; TS for H is 0.13 eV; TS for OH is 0.07 eV; therefore, T∆S is calculated to be 0.148 eV (0.14 eV–0.05 eV + 0.13 eV–0.07 eV = 0.15 eV). Therefore, ∆ZPE - T∆S is −0.18 eV. When the temperature effect of enthalpy is considered, a correction of ΔH should be added [79] , [80] : 
    ΔG=ΔE_DFT+ΔH+ΔZPE-TΔS. (15) 
    Our experiments were conducted at  298K.Therefore, ΔH=H(298K)-H(0K). (16) 
    H(298K)-H(0K)=	H_∗HCO4(298K)-H_HCO3(298K)+0.5H_H2(298K)-H_OH(298K) 
     	 -(H_*HCO4(0K)-H_*HCO3(0K)+0.5H_H2(0K)-H_OH(0K))
 
    =	(H_*HCO4(298K)-H_*HCO4(0K))-(H_*HCO3(298K)-H_*HCO3(0K)) 
     	+0.5(H_H2(298K)-H_H2(0K))-(H_OH(298K)-H_OH(0K))
 
    =C_*HCO4(298K-0K)-C_*HCO3(298K-0K)+0.5C_*H2(298K-0K)-C_OH(298K-0K)
 Where C *HCO4 , C *HCO3 , C *H2 , and C OH is the heat capacity with the unit of J K −1 mol −1 . C *HCO4 , C *HCO3 , C *H2 , and C OH is 39.6, 30.2, 16.6, and 15.9 J K -1 mol -1 , respectively, which are obtained by using the phonopy in VASP. The unit of J K -1 mol -1 is converted to eV by dividing 1.6E-19 and NA (6.02E23 mol -1 ). Finally, the correction of H(298 K) - H(0 K) is calculated to be 0.01 eV. Therefore, at 298 K, the ∆G is calculated to be −1.82 eV (−1.65 eV − 0.18 eV + 0.01 eV) at the potential of 2.3 V versus RHE at 298 K. This negative value suggests that the transformation of *HCO 3 to *HCO 4 on the (311) facet is favorable at 2.3 V versus RHE at 298 K. In the case of the (220) facet, the E *HCO4− E *HCO3 is 0.66 eV; E H is −3.39 eV; E OH is −7.34 eV; U is 2.3 V. Therefore, ∆E is calculated to be 0.01 eV (E *HCO4− E *HCO3 + E H –E OH - 2eU). The ZPE for HCO 3 is 0.66 eV; ZPE for HCO 4 is 0.80 eV; ZPE for H is 0.16 eV; ZPE for OH is 0.33 eV; ∆ZPE is −0.03 eV (0.80 eV- 0.66 eV + 0.16 eV–0.33 eV = 0.03 eV). At 298 K, TS for HCO 3 is 0.05 eV; TS for HCO 4 is 0.14 eV; TS for H is 0.13 eV; TS for OH is 0.07 eV; therefore, T∆S is 0.15 eV (0.14 eV–0.05 eV + 0.13 eV - 0.07 eV = 0.15 eV). Therefore, ∆ZPE–T∆S is −0.18 eV. Therefore, ∆G is calculated to be −0.16 eV at the potential of 2.3 V versus RHE at 298 K. This negative value suggests that at 2.3 V versus RHE the transformation of *HCO 3 to *HCO 4 on (220) facet is favorable. Reporting summary Further information on research design is available in the Nature Portfolio Reporting Summary linked to this article.